Spike timing-dependent selective strengthening of single climbing fibre inputs to Purkinje cells during cerebellar development Shaping functional neural circuits in developing brain involves activity-dependent refinement of early-formed redundant synapses. In the developing cerebellum, a one-to-one connection between a climbing fibre (CF) and a Purkinje cell (PC) is established by selective strengthening of a single CF followed by elimination of surplus CFs. Here we investigate developmental changes in CF-mediated responses in PCs by using in vivo whole-cell recordings and two-photon Ca 2+ imaging. We show that each neonatal PC receives temporally clustered inputs from multiple CFs and temporal integration of these inputs is required to induce burst spiking and Ca 2+ rise in PCs. Importantly, a single CF input closest to PC’s spike output is selectively strengthened during postnatal development. This spike timing-dependent selective strengthening is much less prominent in PC-selective P/Q-type voltage-dependent Ca 2+ channel knockout mice. Thus, spike timing- and Ca 2+ -dependent plasticity appears to underlie the selection of a single ‘winner’ CF and the establishment of mature CF–PC connections. Development of functional neural circuits involves initial formation of supernumerary synaptic connections that is followed by strengthening of necessary synapses and elimination of redundant connections in early postnatal life [1] , [2] , [3] , [4] . Many previous studies demonstrate that neural activity is crucial for these processes [1] , [2] , [3] , [4] . In the developing cerebellum, a one-to-one connection between a climbing fibre (CF) and a Purkinje cell (PC) is established in an activity-dependent manner, which has been a representative case of synapse elimination in the central nervous system (CNS) [5] , [6] , [7] , [8] , [9] . Each PC is innervated by multiple CFs with similar synaptic strengths at birth. From postnatal day 3 (P3) to P7, selective strengthening of a single CF relatively to the other CFs occurs in each PC. Then, the strengthened ‘winner’ CF undergoes translocation to PC dendrites, whereas the ‘loser’ CFs whose synapses are left on the PC soma, are eliminated from P7 to around P17. Thus, the selective strengthening of a single CF from P3 to P7 is crucial for determining the CF that innervates the PC throughout life [10] . In cerebellar slices at P5–9, long-term potentiation (LTP) occurs exclusively at the large CF input, whereas long-term depression (LTD) is induced at the smaller CF inputs, following coincident activation of the CF and depolarization of the PC [11] , [12] . The LTP/LTD at CF to PC synapses is presumed to be a cellular mechanism for promoting the functional differentiation of multiple CFs into a single ‘winner’ CF and ‘loser’ CFs. Recently, we have reported that the functional differentiation of multiple CFs during the first postnatal week is severely impaired in mice with PC-selective deletion of Ca v 2.1, a pore forming subunit of P/Q-type voltage-dependent Ca 2+ channel [13] . This result demonstrates that Ca 2+ influx into PC through P/Q-type Ca 2+ channels mediates synaptic competition among multiple CFs and suggests that Ca 2+ -dependent synaptic plasticity contributes to selective strengthening/weakening of CF inputs during the first postnatal week. However, it is unclear what patterns of activity of CFs and PCs in vivo are correlated with the selective strengthening of single CFs. Investigation of the relationship between CF inputs and PC outputs during development can provide important clues to understand the mechanisms of activity-dependent refinement of CF to PC synapses. In this study, we used in vivo whole-cell patch-clamp recordings [14] , [15] , [16] to investigate synaptic and spiking activities in immature PCs that are relevant to the refinement of CF to PC synapses. We show that temporally clustered excitatory postsynaptic potentials (EPSPs) arising from multiple CF inputs induce burst spiking (BS) in immature PCs. The number of EPSPs preceding BS reflects the number of CFs innervating the PC, both of which decrease with the course of postnatal development. Notably, the amplitude of EPSPs preceding BS is inversely correlated with the interval between the onset of EPSP and BS. Importantly, the EPSP just before the BS selectively becomes larger relatively to the other EPSPs from P4–6 to P7–8. This spike timing-dependent selective strengthening is much less prominent in PC-selective Ca v 2.1 knockout mice than in wild-type mice. Furthermore, our in vivo two-photon Ca 2+ imaging demonstrates that BS is associated with Ca 2+ rise in neonatal PCs whose amplitude is proportional to the number of spikes in BS. These results suggest that the CF synaptic input associated with the initiation of BS and Ca 2+ rise through P/Q-type Ca 2+ channels is selectively strengthened among multiple CF inputs during postnatal development. Burst spiking in immature PCs in vivo In anaesthetised rat from P4 to P17 of age, we performed in vivo whole-cell patch-clamp recordings [14] , [15] , [16] from PCs that were identified by their characteristic electrophysiological and morphological properties ( Fig. 1 , Supplementary Figs S1 and S2 ) [17] , [18] , [19] . Besides ongoing simple spikes (SSs) ( Fig. 1a,c upper traces and Supplementary Fig. S2b ) [7] , [17] , [18] , [20] , [21] , [22] , PCs showed sporadic and oscillatory BS, which consisted of more than two consecutive spikes with <30 ms interspike intervals, in earlier stage of development ( Fig. 1a and Supplementary Fig. S2a ), whereas they showed complex spikes (CSs) in later developmental stages ( Fig. 1c and Supplementary Fig. S2a ). Hyperpolarization of the membrane potential diminished SS, but not BS ( Fig. 1a lower left, b) or CS ( Fig. 1c lower left, d), suggesting that BS and CS are caused by strong synaptic inputs. Interestingly, BS waveforms of PCs in earlier developmental stage showed a higher degree of variability than relatively stable CS waveforms of PCs in later stages ( Fig. 1a right, c right, e–g and Supplementary Fig. S2d,f ). 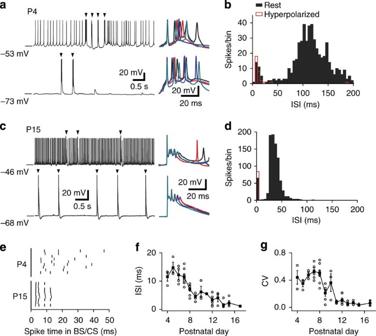Figure 1: Spontaneous firing activities of immature PCs during postnatal development. (a,c) Representative traces of SS and BS/CS (arrowheads) recorded from PCsin vivoat P4 (a) and P15 (c) (upper left). For BS at P4–6, mean occurrence frequency was 0.19±0.05 Hz and mean oscillation frequency was 3.19±0.24 Hz (mean±s.e.m.,n=23). For CS at P14–17, mean occurrence frequency was 0.44±0.07 Hz(mean±s.e.m.,n=11). For SS, mean frequency was 6.5±0.5 Hz at P4–6 (mean±s.e.m.,n=27) and 28.1±6.2 Hz at P14–17(mean±s.e.m.,n=7). SS was suppressed by injecting hyperpolarizing current (lower left). Four BS/CS traces are aligned to the first spike peak and superimposed at resting (upper right) and hyperpolarized potentials (lower right). (b,d) Histograms of interspike interval (ISIH: bin size 5 ms) obtained under resting (black closed bars) and hyperpolarized membrane potentials (red open bars) at P4 (b) and P15 (d) from the same PCs shown in (a) and (c), respectively. The ISIH at rest in earlier stage of development was characterized by two distinguishable peaks, indicating the presence of higher frequency BS (mean ISI in BS: 16.5±0.8 ms, mean±s.e.m.,n=23) and lower frequency SS (b). PCs in later developmental stage also showed two distinguishable peaks in the ISIH, corresponding to SS and spikelets in CS (d). (e) Timing of spikes/spikelets relative to the first spike of BS/CS at P4 (top) and P15 (bottom) for the same PCs shown in (a) and (c), respectively. Note that spikes in BS are more variable than spikelets in CS. (f,g) ISI between the first and second spikes in BS/CS (f) and its coefficient of variation (CV) (g) decreased with age. Open circles represent averaged data for individual cells. Closed squares and error bars represent mean±s.e.m. for the data of each postnatal day. Figure 1: Spontaneous firing activities of immature PCs during postnatal development. ( a , c ) Representative traces of SS and BS/CS (arrowheads) recorded from PCs in vivo at P4 ( a ) and P15 ( c ) (upper left). For BS at P4–6, mean occurrence frequency was 0.19±0.05 Hz and mean oscillation frequency was 3.19±0.24 Hz (mean±s.e.m., n =23). For CS at P14–17, mean occurrence frequency was 0.44±0.07 Hz(mean±s.e.m., n =11). For SS, mean frequency was 6.5±0.5 Hz at P4–6 (mean±s.e.m., n =27) and 28.1±6.2 Hz at P14–17(mean±s.e.m., n =7). SS was suppressed by injecting hyperpolarizing current (lower left). Four BS/CS traces are aligned to the first spike peak and superimposed at resting (upper right) and hyperpolarized potentials (lower right). ( b , d ) Histograms of interspike interval (ISIH: bin size 5 ms) obtained under resting (black closed bars) and hyperpolarized membrane potentials (red open bars) at P4 ( b ) and P15 ( d ) from the same PCs shown in ( a ) and ( c ), respectively. The ISIH at rest in earlier stage of development was characterized by two distinguishable peaks, indicating the presence of higher frequency BS (mean ISI in BS: 16.5±0.8 ms, mean±s.e.m., n =23) and lower frequency SS ( b ). PCs in later developmental stage also showed two distinguishable peaks in the ISIH, corresponding to SS and spikelets in CS ( d ). ( e ) Timing of spikes/spikelets relative to the first spike of BS/CS at P4 (top) and P15 (bottom) for the same PCs shown in ( a ) and ( c ), respectively. Note that spikes in BS are more variable than spikelets in CS. ( f , g ) ISI between the first and second spikes in BS/CS ( f ) and its coefficient of variation (CV) ( g ) decreased with age. Open circles represent averaged data for individual cells. Closed squares and error bars represent mean±s.e.m. for the data of each postnatal day. Full size image To explore the synaptic mechanisms underlying the generation of BS, we observed synaptic inputs in immature PCs in vivo under voltage-clamp mode. At holding potential ( V h ) of −70 mV, PCs showed sporadic and oscillatory burst of excitatory postsynaptic currents (bEPSCs) at around P5 ( Fig. 2a and Supplementary Fig. S3c ). The inter-event interval (IEI) histogram for all EPSCs revealed that majority of IEIs were distributed within 20 ms ( Fig. 2b , black closed bars), and therefore we defined bEPSC as a cluster of more than three consecutive EPSCs with IEI of <20 ms ( Fig. 2b , red open bars). The IEIs of events within individual bEPSCs at P5 were highly variable and showed an exponential distribution ( Fig. 2b , red open bars). In contrast, bEPSCs from PCs at P10 had a single prominent peak in the IEI histogram with much lower variability ( Fig. 2c,d ). Furthermore, the second and later EPSC amplitudes in bEPSC after P10 showed prominent depression, known to be characteristic to CF-PC synapses ( Fig. 2c , right) [23] . This type of bEPSC is similar to the CF burst resulting from the axonal bursts in a single inferior olivary neuron in young rats [24] . We also measured the IEI between the first and the following events in bEPSC. The histogram showed a broad distribution and no sign of specific temporal structure at P5 ( Fig. 2e , upper). By contrast, the histogram at P10 clearly showed distinct narrow peaks that are most likely to correspond to the frequency of burst firing of a single CF ( Fig. 2e , lower). Summary data for IEI and CV of the 1st to 2nd EPSC indicate that the variability of IEI in bEPSC decreased at P10–11 ( Fig. 2f,g and Supplementary Fig. S3d,e ). In addition, the duration and the number of events in bEPSC and their CV decreased with age, also around P10–11 ( Supplementary Fig. S3f–i ). These developmental changes in the variability of bEPSCs were similar to those in BS/CS ( Fig. 1e–g , Supplementary Fig. S2c–f ). These results strongly suggest that BS up to around P10 is generated mainly by multiple CF inputs with variable timings, whereas CS after around P11 is induced by burst firing of a single CF [24] . 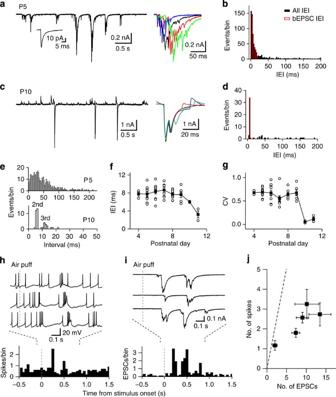Figure 2: Burst excitatory synaptic inputs in immature PCs. (a,c) Spontaneous EPSCs recorded from PCsin vivoat P5 (Vhat −70 mV) (a) and P10 (Vhat −30 mV) (c). Mean occurrence frequency of bEPSCs at P4–6 was 0.22±0.04 Hz (mean±s.e.m.,n=15). On the right, four bEPSC traces are aligned to the first event in each bEPSC and superimposed. Inset in the left panel ofashows the averaged trace of isolated EPSCs. The second and later EPSCs in bEPSC at P10–11 showed prominent depression. The mean value of 2nd EPSC/1st EPSC was 0.34±0.1 (mean±s.e.m.) and that of inter-event interval (IEI) between the 1st and 2nd EPSCs was 4.33±0.81 ms (mean±s.e.m.,n=5). (b,d) Histograms of IEI (bin size: 2.5 ms) obtained from all EPSCs (black closed bars) and EPSCs within each bEPSC (red open bars) at P5 (b) and P10 (d) from the same PCs shown inaandc, respectively. (e) Corresponding histograms of time intervals between the 1st and following EPSCs for cells shown ina(top) andc(bottom), respectively. Note that events in bEPSC at P5 are more variable than P10. (f,g) IEI between the 1st and 2nd events in each bEPSC (f) and its CV (g) decreased with age. Open circles represent averaged data for individual cells. Closed squares and error bars represent mean±s.e.m. for the data of each postnatal day. (h,i) BSs (h) and bEPSCs (i) evoked by sensory stimulation (air puff to the vibrissae or perioral surface) under current-clamp and voltage-clamp modes (Vhat −90 mV), respectively, in a PC at P6 (upper panels). Peristimulus time histograms (lower panels) show clear sensory-evoked responses (bin size: 50 ms). (j) Relationship between the number of sensory-evoked EPSCs and spikes from PCs at P5–6 (n=5). The dashed line indicates the unity line. Each symbol shows data from individual cells. Error bars represent±s.e.m. for individual cells. Figure 2: Burst excitatory synaptic inputs in immature PCs. ( a , c ) Spontaneous EPSCs recorded from PCs in vivo at P5 ( V h at −70 mV) ( a ) and P10 ( V h at −30 mV) ( c ). Mean occurrence frequency of bEPSCs at P4–6 was 0.22±0.04 Hz (mean±s.e.m., n =15). On the right, four bEPSC traces are aligned to the first event in each bEPSC and superimposed. Inset in the left panel of a shows the averaged trace of isolated EPSCs. The second and later EPSCs in bEPSC at P10–11 showed prominent depression. The mean value of 2nd EPSC/1st EPSC was 0.34±0.1 (mean±s.e.m.) and that of inter-event interval (IEI) between the 1st and 2nd EPSCs was 4.33±0.81 ms (mean±s.e.m., n =5). ( b , d ) Histograms of IEI (bin size: 2.5 ms) obtained from all EPSCs (black closed bars) and EPSCs within each bEPSC (red open bars) at P5 ( b ) and P10 ( d ) from the same PCs shown in a and c , respectively. ( e ) Corresponding histograms of time intervals between the 1st and following EPSCs for cells shown in a (top) and c (bottom), respectively. Note that events in bEPSC at P5 are more variable than P10. ( f , g ) IEI between the 1st and 2nd events in each bEPSC ( f ) and its CV ( g ) decreased with age. Open circles represent averaged data for individual cells. Closed squares and error bars represent mean±s.e.m. for the data of each postnatal day. ( h , i ) BSs ( h ) and bEPSCs ( i ) evoked by sensory stimulation (air puff to the vibrissae or perioral surface) under current-clamp and voltage-clamp modes ( V h at −90 mV), respectively, in a PC at P6 (upper panels). Peristimulus time histograms (lower panels) show clear sensory-evoked responses (bin size: 50 ms). ( j ) Relationship between the number of sensory-evoked EPSCs and spikes from PCs at P5–6 ( n =5). The dashed line indicates the unity line. Each symbol shows data from individual cells. Error bars represent±s.e.m. for individual cells. Full size image To quantify the relationship between BS and synaptic inputs, we analysed the sensory-evoked responses in immature PCs ( Fig. 2h–j ). The air puff stimulation to the vibrissae or perioral surface reliably evoked BS ( Fig. 2h ) and bEPSCs ( Fig. 2i ) under current- and voltage-clamp recordings, respectively. We observed no difference between spontaneous and sensory-evoked responses in their basic electrophysiological parameters ( Supplementary Table S1 ). The number of spikes in sensory-evoked BS was consistently smaller than the number of events in sensory-evoked bEPSC in each PC ( n =5 cells at P5–6, Fig. 2j ), implying that temporal clustering of multiple synaptic inputs is required to induce BS. To directly test whether a cluster of synaptic inputs generates BS, we examined spiking activities of PCs by injecting the bEPSC waveforms recorded from the same PCs. This procedure elicited multiple spiking that was indistinguishable from the spontaneous BS ( Fig. 3a–c ). In line with the input–output relationship in sensory-evoked responses ( Fig. 2j ), the number of spikes in the mimicked BS was smaller than the number of events in injected bEPSCs in each PC ( n =4 cells at P5–6, Fig. 3d ). We also found that the area and the number of events in injected bEPSC waveform were strongly correlated with the number of spikes in mimicked BS ( Supplementary Fig. S4a–c ). In contrast, the amplitude of the largest event in injected bEPSC was only weakly correlated with the number of spikes in mimicked BS ( Supplementary Fig. S4d ). On the other hand, currents mimicking single CF-EPSCs injected into PCs at P4–7 could induce multiple spikes only with amplitude much larger (>1 nA, Fig. 3e,f ) than that of the largest EPSC in bEPSCs (109.8±20.83 pA, at P5–6, mean±s.e.m., n =4 cells). Furthermore, the ISI in the BS induced by single-EPSC waveform was significantly shorter than that in spontaneous BS recorded from the same PC ( Fig. 3g,h ). To further confirm that the variability of ISI in BS resulted from the variability of underlying synaptic inputs, we injected the same bEPSC waveforms repeatedly into the same PCs in vivo . The resultant BS exhibited very constant firing patterns, and the timing of each spike in the mimicked BS was significantly more precise than in spontaneous BS recorded from the same PC ( Fig. 3i,j ). All these results indicate that BS is induced by temporally clustered multiple synaptic inputs with variable timings. 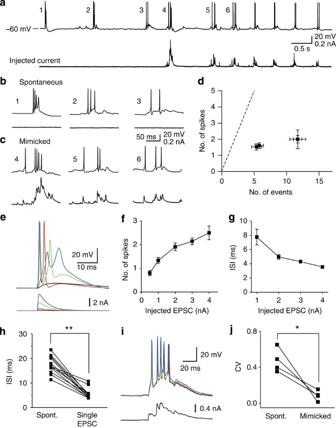Figure 3: BS is mimicked by injecting current waveforms from spontaneous bEPSCs in immature PCs. (a) Spontaneous bEPSCs were transformed into current commands and then these currents (bottom) were injected into the same PC. (b,c) Three examples of spontaneous BS (1–3 ina) were similar to multiple spiking events (4–6 ina) induced by current commands constructed from bEPSCs. (d) Relationship between the number of component EPSCs and spikes in mimicked BSs. The dashed line indicates the unity line. Each symbol shows data from individual cells at P5 and P6 (n=4). Error bars represent±s.e.m. for individual cells. (e) Four voltage traces (upper) evoked by injecting currents mimicking single CF-EPSC waveforms (bottom,t-rise: 0.33 msec,t-decay: 4.48 ms) of increasing intensity into a PC at P5. (f) Averaged number of spikes plotted against current intensities. Error bars represent±s.e.m. for each current intensity. (g) Averaged ISI between the first and second spikes in evoked spikes plotted against current intensities. Error bars represent±s.e.m. for the data obtained at each current intensity. (h) ISI in BS evoked by injecting currents mimicking single EPSC waveforms with peak intensities of 1–4 nA was significantly smaller than that for spontaneous BS (5.56±0.64 ms and 17.4±1.01 ms, respectively at P4–7, mean±s.e.m.,n=12, pairedt-test, **P<0.001). (i) Four mimicked BS traces (upper) evoked by injecting the same bEPSC waveform (bottom) repeatedly. (j) Averaged CV of ISI between the first and second spikes in spontaneous BS and mimicked BS. CV for the mimicked BS was significantly smaller than that for spontaneous BS (0.09±0.03 and 0.47±0.07, respectively at P5–7, mean±s.e.m.,n=4, pairedt-test, *P=0.024). Figure 3: BS is mimicked by injecting current waveforms from spontaneous bEPSCs in immature PCs. ( a ) Spontaneous bEPSCs were transformed into current commands and then these currents (bottom) were injected into the same PC. ( b , c ) Three examples of spontaneous BS (1–3 in a ) were similar to multiple spiking events (4–6 in a ) induced by current commands constructed from bEPSCs. ( d ) Relationship between the number of component EPSCs and spikes in mimicked BSs. The dashed line indicates the unity line. Each symbol shows data from individual cells at P5 and P6 ( n =4). Error bars represent±s.e.m. for individual cells. ( e ) Four voltage traces (upper) evoked by injecting currents mimicking single CF-EPSC waveforms (bottom, t -rise: 0.33 msec, t -decay: 4.48 ms) of increasing intensity into a PC at P5. ( f ) Averaged number of spikes plotted against current intensities. Error bars represent±s.e.m. for each current intensity. ( g ) Averaged ISI between the first and second spikes in evoked spikes plotted against current intensities. Error bars represent±s.e.m. for the data obtained at each current intensity. ( h ) ISI in BS evoked by injecting currents mimicking single EPSC waveforms with peak intensities of 1–4 nA was significantly smaller than that for spontaneous BS (5.56±0.64 ms and 17.4±1.01 ms, respectively at P4–7, mean±s.e.m., n =12, paired t -test, ** P <0.001). ( i ) Four mimicked BS traces (upper) evoked by injecting the same bEPSC waveform (bottom) repeatedly. ( j ) Averaged CV of ISI between the first and second spikes in spontaneous BS and mimicked BS. CV for the mimicked BS was significantly smaller than that for spontaneous BS (0.09±0.03 and 0.47±0.07, respectively at P5–7, mean±s.e.m., n =4, paired t -test, * P =0.024). Full size image Burst inputs from multiple CFs induce BS We found that BS was preceded by several EPSPs at around P6 ( Fig. 4a left, see Supplementary Fig. S5 and Methods for the detection criteria of EPSP events), then BS turned into CS at around P9 ( Fig. 4a centre), and the EPSPs preceding CS subsequently disappeared at around P14 ( Fig. 4a , right). The number of EPSPs preceding BS/CS gradually decreased with the course of development and almost reached the bottom at P11 ( Fig. 4b ). The characteristic waveform of CS, which shows low trial variability ( Fig. 1e,g , Supplementary Fig. S2d,f ), is likely to result from a single strong CF input to that PC. These developmental changes suggest that the transition from immature variable BS to mature stable CS results from strengthening of a single CF and the reduction in the number of CFs innervating individual PCs. 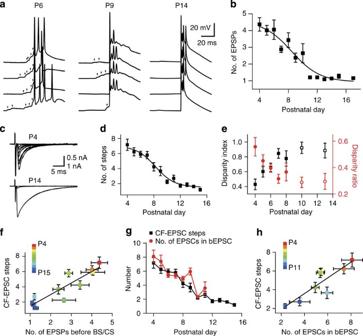Figure 4: Burst EPSPs in immature PCs arise from multiple CF inputs. (a) Representative BS/CS at P6, P9 and P14. Arrowheads indicate EPSPs preceding BS/CS. (b) Averaged number of EPSPs within 50 ms before the BS onset decreased with age. (c) Representative traces showing stepwise recruitments of CF-EPSCs with increasing stimulus intensities at P4 (Vhat −70 mV) and P14 (Vhat −20 mV) in acute cerebellar slices. (d) Developmental change in the averaged number of CF-EPSC steps in PCs (n=5–20) examined in slices. (e) Developmental changes in the disparity index (black) and disparity ratio (red) (n=6–28) obtained from slice experiments. Data for P9–11 and P12–14 are pooled (open symbols). (f) Correlation between the averaged number of CF-EPSC steps examined in slices (data fromd) and the averaged number of EPSPs preceding BS/CS recordedin vivo(data fromb) for postnatal days from P4 to P15. The line is linear fit to data (Pearson’sr=0.9,n=12,t-test,P<0.0001). Postnatal days for individual plotted data are color-coded. (g) Developmental change in the averaged number of CF-EPSC steps (black) (data fromd) and the averaged number of events in bEPSC recordedin vivo(red). (h) Correlation between the averaged number of CF-EPSC steps (data fromd) and the averaged number of events in bEPSC (data fromg) for postnatal days from P4 to P11. The line is linear fit to data (Pearson’sr=0.9,n=8,t-test,P=0.004). Postnatal days for individual plotted data are color-coded. Error bars in (b) and (d–h) represent ±s.e.m. for the data of each postnatal day. Figure 4: Burst EPSPs in immature PCs arise from multiple CF inputs. ( a ) Representative BS/CS at P6, P9 and P14. Arrowheads indicate EPSPs preceding BS/CS. ( b ) Averaged number of EPSPs within 50 ms before the BS onset decreased with age. ( c ) Representative traces showing stepwise recruitments of CF-EPSCs with increasing stimulus intensities at P4 ( V h at −70 mV) and P14 ( V h at −20 mV) in acute cerebellar slices. ( d ) Developmental change in the averaged number of CF-EPSC steps in PCs ( n =5–20) examined in slices. ( e ) Developmental changes in the disparity index (black) and disparity ratio (red) ( n =6–28) obtained from slice experiments. Data for P9–11 and P12–14 are pooled (open symbols). ( f ) Correlation between the averaged number of CF-EPSC steps examined in slices (data from d ) and the averaged number of EPSPs preceding BS/CS recorded in vivo (data from b ) for postnatal days from P4 to P15. The line is linear fit to data (Pearson’s r =0.9, n =12, t -test, P <0.0001). Postnatal days for individual plotted data are color-coded. ( g ) Developmental change in the averaged number of CF-EPSC steps (black) (data from d ) and the averaged number of events in bEPSC recorded in vivo (red). ( h ) Correlation between the averaged number of CF-EPSC steps (data from d ) and the averaged number of events in bEPSC (data from g ) for postnatal days from P4 to P11. The line is linear fit to data (Pearson’s r =0.9, n =8, t -test, P =0.004). Postnatal days for individual plotted data are color-coded. Error bars in ( b ) and ( d – h ) represent ±s.e.m. for the data of each postnatal day. Full size image To test this notion, we examined the time course of the strengthening of a single CF and elimination of surplus CFs in rat cerebellar slices [10] ( Fig. 4c–e , Supplementary Fig. S6 ). The number of CF-EPSC steps in each PC progressively decreased during the second postnatal week ( Fig. 4c,d ). Disparity among the amplitude of CF-EPSC steps in each PC, which reflects the strengthening of a single CF, increased from P4–8 and remained stable thereafter ( Fig. 4e , see Methods for the definition of disparity index and disparity ratio). These results are consistent with the previous reports in mice [10] , [25] and rats [11] that selection of a ‘winner’ CF occurs in the first postnatal week and elimination of supernumerary CFs follows in the second and third postnatal weeks. Importantly, the progressive reduction in the number of EPSPs preceding BS/CS in vivo mirrored the decrease in the number of CF-EPSC steps in a given PC ( Fig. 4b,d,f , Pearson’s r =0.9, n =12, t -test, P <0.0001). We also analysed the developmental change in the number of events in bEPSCs under voltage-clamp mode to determine the total number of inputs in a burst. The number of events in bEPSCs decreased during development, which mirrored the decrease in the number of CF-EPSC steps in cerebellar slices experiments ( Fig. 4g ). It should also be noted that the number of events in bEPSCs in vivo is comparable to the number of CF-EPSC steps in slice ( Fig. 4g,h , Pearson’s r =0.9, n =8, t -test, P =0.004). PCs in early developmental stages are interconnected by their recurrent collaterals [26] , and GABA A receptor (GABA A R)-mediated synaptic inputs can be depolarizing before P10 (refs 26 , 27 ). Therefore, GABA A R-mediated synaptic inputs from neighbouring PCs could contribute to bEPSP/C and BS. To test this possibility, we recorded GABA A R-mediated synaptic currents and their contribution to bEPSCs in immature PCs in vivo . Under voltage-clamp mode at V h of +10 mV, PCs at P6–11 showed spontaneous inhibitory postsynaptic currents (sIPSCs) in vivo ( Supplementary Fig. S7a,b ). Both the frequency and the amplitude of sIPSCs were very low before P8 and increased rapidly from P10 and P9, respectively ( Supplementary Fig. S7c,d ), as previously reported in rats and mice [20] , [27] , [28] , [29] . In the presence of the GABA A R blocker, gabazine (0.4 mM), sIPSC was abolished ( Supplementary Fig. S7e ), but parameters for bEPSC were not altered ( Supplementary Fig. S7f–i ). Therefore, it is unlikely that GABA A R-mediated synaptic inputs from neighbouring PCs contribute to bEPSP/C and the generation of BS. Next, we examined the effects of harmaline ( Fig. 5a–d ), a compound that is known to enhance the synchronous firing of inferior olivary neurons [30] , to further examine the link between bEPSP/C and CF inputs. In rats at P7–9, acute systemic application of harmaline increased the frequency of BS/CS ( Fig. 5a–c ) and EPSP ( Fig. 5d ). Furthermore, chronic injection of harmaline at P9–12 ( Fig. 5e–h ), which has been shown to partially impair CF synapse elimination and increase the number of CFs innervating each PC [31] , increased the average number of EPSPs preceding CS ( Fig. 5g ). In addition, the average amplitude of EPSPs in harmaline-treated rats was larger than that in control rats ( Fig. 5h ). 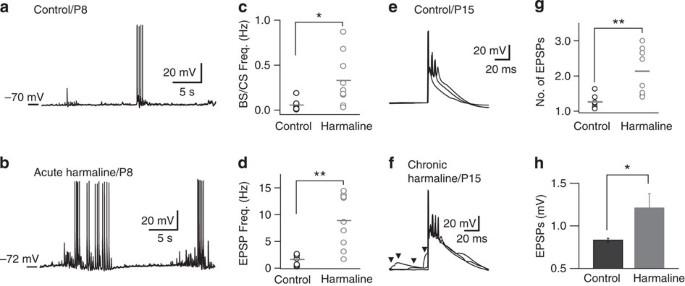Figure 5: Effect of harmaline treatment on immature PCs during postnatal development. (a,b) Membrane potentials of PCs recorded in control (a, saline i.p.) and harmaline (b, 10–30 mg kg−1i.p.)-administered rats with hyperpolarizing current. (c,d) Acute harmaline injection significantly increased the average frequency of BS/CS (c, Mann–WhitneyU-test, *P=0.01) and EPSP (d, Mann–WhitneyU-test, **P=0.002) (control,n=8 from 7 animals; harmaline,n=9 from 8 animals). (e,f) Representative CS recorded in a control rat (e, saline i.p. during P9–12) and that in a rat with chronic treatment of harmaline (f, 30 mg kg−1i.p. during P9–12). Note the EPSPs (arrowheads) preceding CS in the harmaline-treated rat. (g) Number of EPSPs preceding CS (including CS) in harmaline-treated PCs (n=8 from 4 animals at P13–15) was significantly higher than that in control PCs (n=7 in 4 animals at P12–17, Mann–WhitneyU–test, **P=0.002). (h) Averaged amplitude of EPSPs in harmaline-treated PCs was larger than that in control PCs (Mann–WhitneyU-test, *P=0.014). Error bars represent s.e.m. Figure 5: Effect of harmaline treatment on immature PCs during postnatal development. ( a , b ) Membrane potentials of PCs recorded in control ( a , saline i.p.) and harmaline ( b , 10–30 mg kg −1 i.p. )-administered rats with hyperpolarizing current. ( c , d ) Acute harmaline injection significantly increased the average frequency of BS/CS ( c , Mann–Whitney U -test, * P =0.01) and EPSP ( d , Mann–Whitney U -test, ** P =0.002) (control, n =8 from 7 animals; harmaline, n =9 from 8 animals). ( e , f ) Representative CS recorded in a control rat ( e , saline i.p. during P9–12) and that in a rat with chronic treatment of harmaline ( f , 30 mg kg −1 i.p. during P9–12). Note the EPSPs (arrowheads) preceding CS in the harmaline-treated rat. ( g ) Number of EPSPs preceding CS (including CS) in harmaline-treated PCs ( n =8 from 4 animals at P13–15) was significantly higher than that in control PCs ( n =7 in 4 animals at P12–17, Mann–Whitney U –test, ** P =0.002). ( h ) Averaged amplitude of EPSPs in harmaline-treated PCs was larger than that in control PCs (Mann–Whitney U -test, * P =0.014). Error bars represent s.e.m. Full size image Temporally synchronized multiple CF inputs in immature PCs in vivo might also be attributed to the gap junctional coupling between inferior olivary neurons [32] , [33] , [34] (but also refer to the study by Bourrat and Sotelo [35] ). However, acute systemic application of the gap junction blocker carbenoxolone [36] in rats at P6–8 had no effect on the parameters of bEPSC ( Supplementary Fig. S8 ). Thus, gap junctions contribute little, if any, to temporal synchronization of multiple CFs in immature rats. BS induces Ca 2+ transients in immature PCs in vivo While CS is known to generate prominent Ca 2+ transients in mature PCs in vivo [37] , it is unclear whether BS can induce significant Ca 2+ transient in PCs of immature rats. We therefore used the ‘shadowpatching’ technique to make in vivo whole-cell recording and two-photon Ca 2+ imaging from immature PCs with an internal solution containing the Ca 2+ indicator dye Oregon Green 488 BAPTA-1 (refs 14 , 37 ) ( Fig. 6a ). Clear Ca 2+ transients were induced by BS in immature PCs in vivo ( Fig. 6b ), indicating that postsynaptic Ca 2+ elevation coincides with presynaptic CF activity. We found that the amplitude of Ca 2+ transient was proportional to the number of spikes in BS ( Fig. 6c,d ). SS-triggered average of Ca 2+ transients also showed detectable Ca 2+ elevation by each SS ( Fig. 6e ). However, the amplitude of Ca 2+ transients induced by SS was significantly smaller than that by BS, even compared with that triggered by single spikes in BS ( Fig. 6f ). These results indicate that BS triggers large Ca 2+ influx over the baseline Ca 2+ level that is maintained by ongoing SS. The reason why the amount of Ca 2+ influx into PCs triggered by single spikes in BS is larger than that by SS is unclear. The Ca 2+ influx though NMDA receptor (NMDAR) might be involved, because the NMDAR is well known as a coincidence detector for spike timing-dependent plasticity (STDP) [38] . In cerebellar PCs, NMDARs including GluN2D subunit are expressed transiently during early postnatal development at least until P10 (ref. 39 ). However, a previous report has shown that neither CF-EPSC nor CF-LTP could be affected by NMDAR blockers, and no NMDAR-mediated synaptic currents were observed [11] . Therefore, we examined whether NMDAR contributes to Ca 2+ transients triggered by multiple CF inputs in immature PCs at P7–9 in rat cerebellar slices. We found that Ca 2+ transients in PCs triggered by spiking following stimulation of multiple CFs were not affected by either R -CPP (a potent NMDAR blocker) or PPDA (a highly specific blocker against GluN2C/D-containing NMDARs [40] ) ( Supplementary Fig. S9 ). This result confirmed that NMDARs have little, if any, contribution to CF-mediated synaptic responses in immature PCs and suggests that the maturation of CF is independent of NMDAR activity. 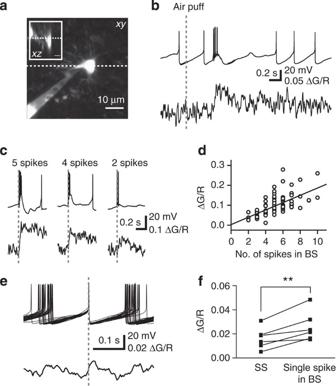Figure 6: BS induces Ca2+transients in immature PCs. (a)xyandxz(inset) projections of the image stack of a recorded PC (P6). Dashed lines indicate locations of line scan. (b) Sensory-evoked BS (top) and simultaneously recorded Ca2+transient (bottom) in the PC shown ina. (c) Representative Ca2+transients (bottom) induced by BS with 5, 4 or 2 spikes (top). Dashed line indicates the time point of the first spike in BS. (d) The amplitude of BS-triggered Ca2+transients was dependent on the number of spikes in BS (open circles,n=91, from six cells, P6–9). Lines are linear fit to the data (Pearson’sr=0.63,t-test,P<0.0001). (e) Overlay of 30 consecutive SS traces (upper) and the averaged Ca2+transient (bottom) triggered by these SSs. (f) Comparison within individual PCs between the averaged amplitude of Ca2+transients triggered by SSs and that by single spikes in BS estimated as (the amplitude of BS-triggered Ca2+transients)/(the number of spikes in BS). The amplitude of Ca2+transients elicited by a single spike in BS was significantly larger than that triggered by a SS (n=6, pairedt-test,P=0.008). Figure 6: BS induces Ca 2+ transients in immature PCs. ( a ) xy and xz (inset) projections of the image stack of a recorded PC (P6). Dashed lines indicate locations of line scan. ( b ) Sensory-evoked BS (top) and simultaneously recorded Ca 2+ transient (bottom) in the PC shown in a . ( c ) Representative Ca 2+ transients (bottom) induced by BS with 5, 4 or 2 spikes (top). Dashed line indicates the time point of the first spike in BS. ( d ) The amplitude of BS-triggered Ca 2+ transients was dependent on the number of spikes in BS (open circles, n =91, from six cells, P6–9). Lines are linear fit to the data (Pearson’s r =0.63, t -test, P <0.0001). ( e ) Overlay of 30 consecutive SS traces (upper) and the averaged Ca 2+ transient (bottom) triggered by these SSs. ( f ) Comparison within individual PCs between the averaged amplitude of Ca 2+ transients triggered by SSs and that by single spikes in BS estimated as (the amplitude of BS-triggered Ca 2+ transients)/(the number of spikes in BS). The amplitude of Ca 2+ transients elicited by a single spike in BS was significantly larger than that triggered by a SS ( n =6, paired t -test, P =0.008). Full size image Spike timing-dependent strengthening of a single CF input Synchronous inputs from multiple CFs that produce BS and Ca 2+ rise in immature PCs ( Fig. 6 ) are well suited to induce spike timing-dependent LTP/LTD, which is considered to underlie selective strengthening/weakening, respectively, of developing synapses [41] . To directly explore the relationship between synaptic strengthening and the timing of CF inputs, we plotted the amplitude of each component EPSP preceding BS against the interval between the onset of component EPSP and BS ( Fig. 7a,b ). We found a strong inverse correlation between these two parameters ( Fig. 7c ). Importantly, the averaged amplitude of EPSP just before BS onset selectively became larger during development ( Fig. 7c ). The largest events were distributed most frequently around BS in both developmental stages ( Supplementary Fig. S10a,b ). Moreover, there was a strong inverse correlation between the amplitude of component EPSP and its timing relative to the onset of the largest EPSP ( Supplementary Fig. S10c ). It should be noted that only the largest EPSP became larger during development (‘interval 0’ in Supplementary Fig. S10c ). These results strongly suggest that the CF input just before the onset of BS is selectively strengthened. However, under current-clamp mode, it was difficult to measure correctly the amplitude of EPSP preceding BS because of spike generation. Therefore, we recorded bEPSCs under voltage-clamp mode and examined the correlation between the amplitude of component EPSC and its timing relative to the largest component EPSC in each bEPSC ( Fig. 7d–f ). We found that the amplitude of component EPSC was inversely correlated with the interval between the component EPSC and the largest EPSC ( Fig. 7d–f ). This inverse correlation is similar to that observed for EPSPs under current-clamp mode ( Fig. 7c ). Furthermore, the amplitude of component EPSC relative to that of the largest EPSC became significantly smaller with age ( Fig. 7f ), indicating that the disparity between the largest EPSC and the other component EPSCs became larger with age. The amplitude ratio of component EPSC to the largest EPSC is comparable to the disparity ratio obtained from the slice experiments ( Fig. 7g , see also Fig. 4e ) and the CV of EPSC amplitudes in each bEPSC is comparable to the disparity index obtained from the slice experiments ( Fig. 7h , see also Fig. 4e ). As the timing of the largest EPSC is most likely to correspond to the onset of BS, we injected bEPSC waveform into immature PCs under current-clamp mode, and analysed the relationship between the amplitude of component EPSC and its timing to the onset of the mimicked BS ( Supplementary Fig. S11a,b ). The amplitude of EPSC was largest at the onset of BS ( Supplementary Fig. S11c ), suggesting that the largest EPSC initiates BS. Thus, these results collectively indicate that a single CF input is selectively strengthened in each PC depending on its input timing relative to BS. 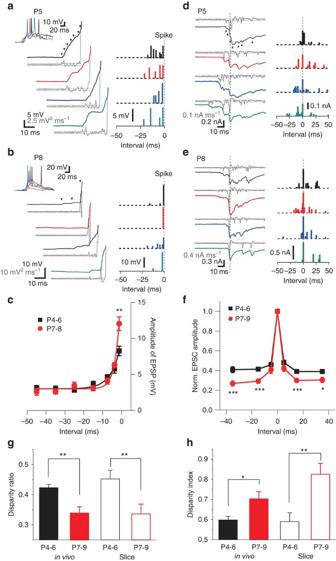Figure 7: Spike timing-dependent strengthening of a ‘winner’ CF. (a,b) Four representative spontaneous BSs at P5 (a) and P8 (b) are superimposed (left, top). EPSPs preceding BS (coloured thick lines) and the second derivative of membrane potential (grey thin lines) are shown on an expanded time scale (left, lower traces). Arrowheads indicate the peaks of individual events. Dashed lines attached to the traces of the second derivative represent±3 s.d. of the baseline noise. Amplitudes of EPSPs are plotted against the interval from the first spike in BS (right). Note that amplitudes of EPSPs clearly decreased as the interval increased. (c) Summary graph showing the relationship between the amplitude of EPSPs and its timing to the onset of BS at P4–6 (black,n=12) and P7–8 (red,n=17) (bin width: 2.5 ms for 0–5 ms, 5 ms for 5–10 ms, 10 ms for 10–50 ms). The averaged amplitude of EPSP at the first bin (0–2.5 ms) in P7–8 was significantly larger than that in P4–6 (n=12 at P4-6,n=17 at P7-8,t-test, **P=0.006). (d,e) Four representative spontaneous bEPSCs (coloured thick lines) and the first derivative of membrane current (grey thin lines, dashed lines represent±3 s.d. of the baseline noise.) (left).Vhwas −70 mV for P5 indand −40 mV for P8 ine. Arrowheads indicate the peaks of individual events. Amplitudes of component EPSCs are plotted against the interval from the largest EPSC in each bEPSC (right). Amplitudes of component EPSCs clearly decreased as the interval increased. (f) Summary graph of normalized EPSC amplitudes plotted against the interval at P4–6 (n=17) and P7–9 (n=22) (bin width: 10 ms for±0–20 ms, 30 ms for±20–50 ms). The values for ±10–20 ms and ±20–50 ms at P7–9 were significantly smaller than those at P4–6 (t-test for +30–50 ms bin and +10–20 ms bin, Mann–WhitneyU-test for −10–20 ms bin and −30–50 ms bin, *P=0.013, ***P<0.001). (g,h) Developmental changes in the disparity ratio (g) and index (h) calculated from spontaneous bEPSCsin vivo(Disparity ratio:t-test,P=0.002, index: Mann-Whitney U test,P=0.04) and CF-EPSC steps recorded in acute cerebeller slices (Disparity ratio:t-test,P=0.01, index:t-test,P=0.002, data fromFig. 4e). Error bars in (c) and (f–h) represent s.e.m. Figure 7: Spike timing-dependent strengthening of a ‘winner’ CF. ( a , b ) Four representative spontaneous BSs at P5 ( a ) and P8 ( b ) are superimposed (left, top). EPSPs preceding BS (coloured thick lines) and the second derivative of membrane potential (grey thin lines) are shown on an expanded time scale (left, lower traces). Arrowheads indicate the peaks of individual events. Dashed lines attached to the traces of the second derivative represent±3 s.d. of the baseline noise. Amplitudes of EPSPs are plotted against the interval from the first spike in BS (right). Note that amplitudes of EPSPs clearly decreased as the interval increased. ( c ) Summary graph showing the relationship between the amplitude of EPSPs and its timing to the onset of BS at P4–6 (black, n =12) and P7–8 (red, n =17) (bin width: 2.5 ms for 0–5 ms, 5 ms for 5–10 ms, 10 ms for 10–50 ms). The averaged amplitude of EPSP at the first bin (0–2.5 ms) in P7–8 was significantly larger than that in P4–6 ( n =12 at P4-6, n =17 at P7-8, t -test, ** P =0.006). ( d , e ) Four representative spontaneous bEPSCs (coloured thick lines) and the first derivative of membrane current (grey thin lines, dashed lines represent±3 s.d. of the baseline noise.) (left). V h was −70 mV for P5 in d and −40 mV for P8 in e . Arrowheads indicate the peaks of individual events. Amplitudes of component EPSCs are plotted against the interval from the largest EPSC in each bEPSC (right). Amplitudes of component EPSCs clearly decreased as the interval increased. ( f ) Summary graph of normalized EPSC amplitudes plotted against the interval at P4–6 ( n =17) and P7–9 ( n =22) (bin width: 10 ms for±0–20 ms, 30 ms for±20–50 ms). The values for ±10–20 ms and ±20–50 ms at P7–9 were significantly smaller than those at P4–6 ( t -test for +30–50 ms bin and +10–20 ms bin, Mann–Whitney U -test for −10–20 ms bin and −30–50 ms bin, * P =0.013, *** P <0.001). ( g , h ) Developmental changes in the disparity ratio ( g ) and index ( h ) calculated from spontaneous bEPSCs in vivo (Disparity ratio: t -test, P =0.002, index: Mann-Whitney U test, P =0.04) and CF-EPSC steps recorded in acute cerebeller slices (Disparity ratio: t -test, P =0.01, index: t -test, P =0.002, data from Fig. 4e ). Error bars in ( c ) and ( f – h ) represent s.e.m. Full size image Importance of P/Q-type voltage-dependent Ca 2+ channel in PC Recently, we have shown that functional differentiation of multiple CFs during the first postnatal week is severely impaired in mice with PC-selective deletion of Ca v 2.1, a pore-forming subunit of P/Q-type voltage-dependent Ca 2+ channel (PC-Ca v 2.1 KO mice) [13] . Therefore, if the spike timing-dependent selective strengthening of single CF underlies the functional differentiation of multiple CFs, it should be impaired in PC-Ca v 2.1 KO mice. We found that spontaneous BS/CS were preceded by several EPSPs in both PC-Ca v 2.1 KO mice and wild-type littermates (control), and the amplitude of EPSP preceding BS/CS were inversely correlated with the interval between each component EPSP and to the onset of BS ( Fig. 8a,b ). Importantly, the averaged amplitude of EPSP just before the BS/CS onset was significantly smaller in PC-Ca v 2.1 KO mice than in control mice, whereas other EPSPs with longer intervals in PC-Ca v 2.1 KO mice had similar amplitudes to those in control mice ( Fig. 8c ). Furthermore, we recorded bEPSCs under voltage-clamp mode and examined the correlation between the amplitude of component EPSC and its timing relative to the largest component EPSC in each bEPSC ( Fig. 8d–f ). We found that the amplitude of component EPSC was inversely correlated with the interval between the component EPSC and the largest EPSC in both control and PC-Ca v 2.1 KO mice ( Fig. 8d,e ). Importantly, the amplitude of component EPSC relative to that of the largest EPSC was significantly larger in PC-Ca v 2.1 KO mice than in control mice ( Fig. 8f,g left), indicating that the disparity between the largest EPSC and the other component EPSCs in PC-Ca v 2.1 KO was smaller than that of control mice. The CV of EPSC amplitudes in each bEPSC is comparable to the disparity index obtained from the previous slice experiments ( Fig. 8g , left) [13] . Moreover, the total amplitude of bEPSC (that is, the sum of the amplitudes of all component EPSCs in bEPSC) was not different between control and PC-Ca v 2.1 KO mice, which is consistent with the data from the previous slice experiments ( Fig. 8g right) [13] . These results demonstrate that PC-Ca v 2.1 KO mice are severely impaired in spike timing-dependent strengthening of a single CF input. Taken together, our results ( Figs 7 and 8 ) support that the strengthening of a ‘winner’ CF may be driven by STDP that is mediated by P/Q-type voltage-dependent Ca 2+ channel in PCs. The degree of synchrony among multiple CF inputs is considered to be important for fine control of plasticity at CF-PC synapses. 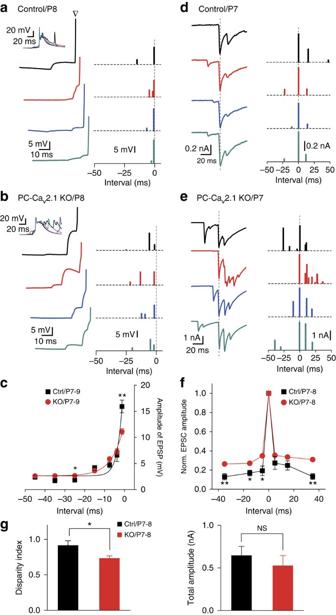Figure 8: Impaired spike timing-dependent strengthening of a ‘winner’ CF in PC-Cav2.1 KO mice. (a,b) Four representative spontaneous BS/CSs in control mouse at P8 (a) and PC-Cav2.1 KO mouse at p8 (b) were superimposed (left, top). EPSPs preceding BS/CS are shown on an expanded time scale (left, lower traces). The average number of EPSPs at P7–9 was 1.89±0.12 for PC-Cav2.1 KO mice (mean±s.e.m.,n=11) and 1.61±0.18 for control mice (mean±s.e.m.,n=8) with no significant difference (t-test,P=0.199). Amplitudes of EPSPs are plotted against the interval from the first spike in BS (right). The amplitude of EPSP inducing CS was determined as the height from baseline to action potential threshold (open arrowhead ina). (c) Summary graph showing the relationship between the amplitude of EPSPs and its timing to the onset of BS in control (n=8, P7–9) and PC-Cav2.1 KO mice (n=11, P7–9) (bin width: 2.5 ms for 0–5 ms, 5 ms for 5–10 ms, 10 ms for 10–50 ms). The averaged amplitude of EPSP at the first bin (0–2.5 ms) in PC-Cav2.1 KO mice (n=11) was significantly smaller than that in control (n=8) (Mann–WhitneyU-test, **P=0.006). (d,e) Four representative spontaneous bEPSCs (left).Vhwas −20 mV in control mice at P7 (d) and −50 mV in PC-Cav2.1 KO mice at P7 (e). Amplitudes of component EPSCs are plotted against the interval from the largest EPSC in each bEPSC (right). (f) Summary graph of normalized EPSC amplitudes plotted against the interval in control and PC-Cav2.1 KO mice (n=11 andn=9, respectively at P7–8,t-test, *P<0.03, **P<0.006). (g) The difference in the disparity index (left,t-test, *P=0.041) and the total amplitude of bEPSC (right, amplitudes at −20 mV were obtained assuming that the current–voltage relationship of EPSC is linear, Mann–WhitneyU-test,P=0.4) calculated from spontaneous bEPSCin vivobetween control and PC-Cav2.1 KO mice. Error bars in (c), (f) and (g) represent s.e.m. Figure 8: Impaired spike timing-dependent strengthening of a ‘winner’ CF in PC-Ca v 2.1 KO mice. ( a , b ) Four representative spontaneous BS/CSs in control mouse at P8 ( a ) and PC-Cav2.1 KO mouse at p8 ( b ) were superimposed (left, top). EPSPs preceding BS/CS are shown on an expanded time scale (left, lower traces). The average number of EPSPs at P7–9 was 1.89±0.12 for PC-Ca v 2.1 KO mice (mean±s.e.m., n =11) and 1.61±0.18 for control mice (mean±s.e.m., n =8) with no significant difference ( t -test, P =0.199). Amplitudes of EPSPs are plotted against the interval from the first spike in BS (right). The amplitude of EPSP inducing CS was determined as the height from baseline to action potential threshold (open arrowhead in a ). ( c ) Summary graph showing the relationship between the amplitude of EPSPs and its timing to the onset of BS in control ( n =8, P7–9) and PC-Ca v 2.1 KO mice ( n =11, P7–9) (bin width: 2.5 ms for 0–5 ms, 5 ms for 5–10 ms, 10 ms for 10–50 ms). The averaged amplitude of EPSP at the first bin (0–2.5 ms) in PC-Ca v 2.1 KO mice ( n =11) was significantly smaller than that in control ( n =8) (Mann–Whitney U -test, ** P =0.006). ( d , e ) Four representative spontaneous bEPSCs (left). V h was −20 mV in control mice at P7 ( d ) and −50 mV in PC-Ca v 2.1 KO mice at P7 ( e ). Amplitudes of component EPSCs are plotted against the interval from the largest EPSC in each bEPSC (right). ( f ) Summary graph of normalized EPSC amplitudes plotted against the interval in control and PC-Ca v 2.1 KO mice ( n =11 and n =9, respectively at P7–8, t -test, * P <0.03, ** P <0.006). ( g ) The difference in the disparity index (left, t -test, * P =0.041) and the total amplitude of bEPSC (right, amplitudes at −20 mV were obtained assuming that the current–voltage relationship of EPSC is linear, Mann–Whitney U -test, P =0.4) calculated from spontaneous bEPSC in vivo between control and PC-Ca v 2.1 KO mice. Error bars in ( c ), ( f ) and ( g ) represent s.e.m. Full size image We demonstrated that characteristic BS in immature rat PCs in vivo was caused by temporally clustered multiple CF inputs. Although the firing of PCs that is analogous to BS and clearly distinct from SS has been reported in immature PCs [17] , [28] , it has been unclear what pattern of CF synaptic inputs underlies BS. The results of the present study clearly indicate that BS in immature PCs is not induced by a single CF input but by temporally clustered excitatory synaptic inputs from multiple CFs. The present results also suggest that highly variable waveforms of BS in immature PCs are primarily attributable to the variety of temporal pattern of multiple CF inputs. High-frequency burst firing of single CFs [24] , [42] becomes apparent after the strengthening of a single CF in each PC ( Fig. 2c,d ). It has been shown that high-threshold Ca 2+ spikes, which are thought to be the source of axonal burst in inferior olivary neuron [24] , are rarely observed in immature inferior olivary neurons until about the end of the first postnatal week [43] . Therefore, high-frequency burst firing of single CFs seems to contribute little, if any, to the generation of BS. In mature animals, inferior olivary neurons, which give rise to CFs, are electrically coupled by gap junctions [44] , [45] , [46] . This coupling is known to underlie synchronous firing of CSs in neighbouring PCs [32] , [33] , [34] . In paired extracellular unit recordings from PCs in immature rat cerebellum, highly synchronized CF responses between nearby PCs has been observed, and the degree of synchrony is higher than that in mature rats [47] . Therefore, the temporally clustered multiple CF inputs that we observed in immature PCs are likely to be attributable in part to the highly synchronized firing of inferior olivary neurons. This enhanced synchrony between immature PCs is supposed to be attributable to weak inhibitory synaptic transmission in the inferior olive, which results in enhanced electrical coupling by gap junctions between neurons [47] . However, the expression level of connexin 36, a dominant subtype of connexin that constitute gap junctions in the inferior olive, is lower in immature mice than in the adult [48] . Moreover, in an electron microscopic study, neuronal gap junctions in the medial accessory olive of rat were not detected until P10 (ref. 35 ). In the present study, we found no effect of gap junction blocker carbenoxolone on parameters of bEPSCs ( Supplementary Fig. S8 ). These results suggest that factors other than gap junctions, presumably chemical synaptic transmissions that are known to exist in the inferior olive before the appearance of gap junctions [35] , [43] , contribute to the enhanced synchrony between inferior olivary neurons at early postnatal development. In addition to the synchrony in the inferior olive, innervation pattern of PCs by CFs in the cerebellar cortex should be important for temporal clustering of EPSPs. Morphological studies show that ‘creeper–type’ CFs innervate the PC soma in early postnatal days, and the number of CFs originating from single olivary axon was >100, which is much larger than that (~7) in the adult [49] . This result indicates that on average >14 CFs innervate a single PC [49] . Burst inputs composed of >10 excitatory synaptic events were often observed ( Figs 2a , 3c and 7d ). Therefore, it is most likely that synchronous firing in multiple inferior olivary neurons transmit their activities to the same PC through CFs and induce bEPSPs in immature cerebellum. Recent electrophysiological and anatomical studies have revealed that there are four distinct stages in the maturation of CF to PC synapses [10] , [25] , [50] , [51] . (1) ‘Functional differentiation of multiple CFs’ occurs from P3 to P7 in which disparity among the strengths of multiple CF inputs in each PC becomes progressively larger from P3 to P6 and reaches a plateau at P7 in mice [10] and rats ( Fig. 4e ). (2) ‘CF translocation to PC dendrites’ is the phenomenon that the strengthened single CF extends its innervation to PC dendrites, which starts at P9 and continues until the fourth postnatal week in mice [25] . (3) ‘Early phase of CF elimination’ occurs from P7 to around P11, which is independent of synapse formation onto PCs from parallel fibres (PFs), the other excitatory input to PCs [50] . (4) ‘Late phase of CF elimination’ proceeds from around P12 to P17 and requires proper formation of PF to PC synapses [50] . We found that EPSPs preceding BS/CS became undetectable at around P11 in PCs in vivo , which is likely to reflect the results of ‘functional differentiation of multiple CFs’ from P3 to P7 and ‘early phase of CF elimination’ from P7 to P11. On the other hand, transition from BS to CS, which occurs in the second postnatal week ( Fig. 4a ), is considered to correspond to the beginning of dendritic translocation of a single ‘winner’ CF as well as the ‘early phase of CF elimination’. The temporal clustering of multiple CF inputs, which is required for the generation of BS, appears to facilitate homosynaptic competition among multiple CFs in individual PCs. Contribution of PF inputs to BS should be negligible particularly before P6. Immunohistochemical analyses have revealed that immature PF varicosities in the molecular layer, which express both VGluT1 and VGluT2, are almost undetectable before P6 and first appear at P7 in the mouse cerebellum [52] , [53] . Consistent with these observations, both in vivo and in vitro electrophysiology has revealed that PF-mediated responses were observed in PCs only after P7 (refs 53 , 54 ). In addition, it has recently been shown that a fraction of mossy fibres (MFs), the other glutamatergic afferent to the cerebellum, can transiently form direct synaptic contacts onto PCs until the second postnatal week [55] . As only a minor fraction of PCs (<30%) are innervated by MFs, it is unlikely that these MF inputs have a major role in bEPSPs. In addition to the glutamatergic synapses, GABAergic synapses also exist onto PCs in developing mice cerebellum and have important roles in the activity and maturation of cerebellar network. It has been reported that depolarizing GABAergic synapses between interconnected PCs generate travelling waves of activity in PCs [26] . Inhibitory synaptic connections from molecular layer interneurons to PCs are involved in the regulation of CF synapse elimination after P10 in mice [27] . However, we observed only low-frequency and small-amplitude IPSCs before P9, and the GABA A R blocker did not alter parameters of bEPSCs recorded in PCs at P5–8 ( Supplementary Fig. S7 ). These results indicate that GABAergic inputs are not involved in the generation of bEPSCs before P9. In vivo two-photon Ca 2+ imaging of immature PCs clearly shows that BS triggered by multiple CF inputs induces Ca 2+ transients in PCs, whereas SS causes Ca 2+ transients that are significantly smaller than those by single spikes in BS ( Fig. 6 ). The competition among multiple CFs is expected to be mediated by Ca 2+ -dependent signalling cascades in PCs. In support of this notion, global and PC-selective deletions of P/Q-type VDCC in mice [13] , [56] are reported to delay selective strengthening of single CFs and to impair early phase of CF synapse elimination and to permit multiple CFs to undergo translocation to PC dendrites. Moreover, it has been shown that LTP/LTD of CF to PC synapses is determined by the amplitude of CF-mediated EPSC, that is, LTP is induced in large CF-mediated EPSP/Cs and LTD occurs in small EPSCs [11] , [12] . It has also been shown that this LTP at CF-PC synapses is dependent on the level of Ca 2+ transients in PCs. Therefore, it is possible that Ca 2+ influx through P/Q-type VDCCs in PCs during BS may trigger LTP, which in turn leads to differentiation into a single ‘winner’ CF and the rest of ‘loser’ CFs. We demonstrated that amplitude of component EPSPs was inversely correlated with the interval between the EPSP and the BS onset ( Figs 7a–c and 8a–c ). Importantly, the difference in averaged amplitude of EPSPs just before the onset of BS became larger from P4–6 to P7–8 ( Fig. 7c ). Furthermore, we found a similar inverse correlation between the amplitude of component EPSC and its timing relative to the largest component EPSC in each bEPSC under voltage-clamp mode ( Figs 7d–f and 8d–f ). This tendency became more prominent from P4–6 to P7–9 ( Fig. 7f ). As the timing of the largest EPSC corresponded to the onset of BS ( Supplementary Fig. S11 ), these results suggest that the EPSP/C associated with the initiation of BS selectively strengthened with development. Induction of LTP/LTD at the CF-PC synapse in slices from P6–9 rats does not depend on the timing between CF input and postsynaptic depolarization but directly to the strength of the CF input [11] . Our results suggest that the strengthening of the largest CF depends on the timing between CF input and BS in PCs. However, we did not observe weakening of smaller CF inputs ( Fig. 7c ). Further investigation will be required to elucidate the cellular mechanisms underlying the weakening of smaller CFs. Furthermore, as multiple CFs innervating a PC have similarly weak synaptic strengths at the earliest postnatal age in mice [10] and rats ( Fig. 4e ), the amplitude-dependent bidirectional plasticity of immature CF [11] , [12] cannot fully explain the mechanisms of the selective strengthening of a single CF at the very beginning of the development. Some additional mechanisms should be considered for the initiation of the functional differentiation among multiple CFs. Impairment of functional differentiation in PC-Ca v 2.1 KO mice in vivo ( Fig. 8c,f ) suggests that the Ca 2+ -dependent synaptic plasticity contributes to selective strengthening/weakening of CF inputs during the first postnatal week. Thus, it is legitimate to assume that spike timing- and Ca 2+ -dependent plasticity underlies selective strengthening of a single CF among multiple CFs in each PC during the first postnatal week. Temporally clustered multiple CF inputs are important for the generation of BS and provide the chance of coincidence between a particular CF input and Ca 2+ transients in PCs. It should be noted that weak CFs are not simply ‘losers’ but can contribute to the generation of BS by firing in cluster with strong CF inputs and thus can promote the selection of a single ‘winner’ CF. In vivo whole-cell patch-clamp recordings All experiments were conducted according to the national guidelines and approved by the Animal Experiment Committees of The University of Tokyo and Hiroshima University. Male and female juvenile Sprague-Dawley rats (P4–17), PC-Ca v 2.1 KO mice and their control littermates (P7–9) [13] , and C57BL/6 mice (P7–8, used as control for voltage-clamp recordings shown in Fig. 8d–f ) were used. Animals were anaesthetised with isoflurane (2–4%). The depth of anaesthesia was monitored by vibrissae movements and withdrawal reflex to hindlimb pinch. Body temperature was maintained at 37±1 °C using a heating pad (BRC). The animal’s head was fixed on a stereotaxic apparatus with ear bars (Narishige). After cutting the skin and removing muscles and connective tissues, the skull over the cerebellum was exposed. Lidocaine gel was applied to the skin incision. A craniotomy (2–3 mm in diameter) was performed by using a micro-drill (NSK) to expose a cerebellar folium (Crus II of the hemisphere or lobule 6 and 7 of the vermis). Subsequently, the dura was cut using a 30G syringe needle and fine forceps. The craniotomy was then filled with 1.5% low-melting point agarose dissolved in HEPES-buffered saline containing (in mM): 150 NaCl, 2.5 KCl, 10 HEPES, 2 CaCl 2 , 1 MgCl 2 (pH 7.3). Whole-cell patch-clamp recordings were made with a Multiclamp 700B amplifier (Molecular Devices) by in vivo blind patch-clamp techniques [16] . In brief, a high positive pressure (100–200 mbar) was applied to the pipette to prevent tip occlusion while penetrating the agarose and the pia. After passing the pia, the positive pressure was immediately reduced (25–35 mbar) to prevent cortical damage. The pipette was advanced by 2 μm steps, and target cells were searched by monitoring the pipette resistance under voltage-clamp mode with a square voltage step (10 mV, 20 ms duration at 50 Hz). When the current pulse amplitude decreased suddenly (20–50%), quick removal of the positive pressure (following gentle suction, if required to obtain tight seals) resulted in a gigaohm seal (>1 GΩ). After cell-attached configuration, whole-cell configuration was obtained by breaking the patch membrane using a slow ramp of negative pressure. The resistance of the patch pipette was 5–10 MΩ when filled with one of the internal solutions with the following compositions (in mM): (1) 133 KMeSO 3 , 7.4 KCl, 10 HEPES, 3 Na 2 ATP, 0.3 Na 2 GTP, 0.3 MgCl 2 , 0.05–0.1 EGTA, pH 7.3; (2) same as the solution (1) but contained 5 QX314; (3) 132 CsMeSO 3 , 10 HEPES, 3 Na 2 ATP, 0.3 Na 2 GTP, 0.3 MgCl 2 , 1 EGTA, 5 QX314, pH 7.3. The internal solution (1) was for all current-clamp experiments and voltage-clamp experiments in PCs at P4–6, whereas the solutions (2) and (3) were used in voltage-clamp experiments for PCs at P7–11. The solution (3) was used for voltage-clamp experiments shown in Supplementary Figs S7 and S8 . Liquid junction potential (+10 mV) was not corrected. Low-chloride internal solution was used to separate glutamatergic EPSCs and GABA A receptor-mediated IPSCs. Series resistance was typically 20–100 MΩ in current-clamp experiments and 20–50 MΩ in voltage-clamp experiments. Our voltage-clamp recordings had sufficient sensitivity to detect unitary EPSCs at V h of −70 mV ( Fig. 2a inset, 10–90% rise time=1.19±0.07 ms, mean±s.e.m. ; decay time=6.1±0.5 ms, mean±s.e.m., at P4–8, n =19) and unitary IPSCs at V h of +10 mV ( Supplementary Fig. S7a,b , 10–90% rise time=2.38±0.93 ms, mean±s.e.m. ; decay time=22.91±6.66 ms, mean±s.e.m., at P6–11, n =17). Electrophysiological data were filtered at 3 or 10 kHz and digitized at 20 kHz with an ITC-16 interface (Instrutech), and acquired with Axograph X software (Axograph Scientific). Data were analysed with Axograph X, Excel (Microsoft) and OriginPro (OriginLab). PCs were identified by their larger capacitance, lower input resistance, presence of a stronger sag ( I h ) and characteristic spontaneous firing patterns composed of both SS and BS/CS, which were distinguishable from other cell-types ( Fig. 1 , Supplementary Figs S1 and S2 ) [19] , [57] . Spiking events and postsynaptic potentials or currents were automatically detected and analysed by MiniAnalysis Program (Synaptosoft). Isolated EPSCs/IPSCs were detected as non-overlapping events within 30 or 50 ms of event intervals for EPSCs or IPSCs respectively. Their parameters (10–90% rise and t -decay) were calculated from averaged traces in each cell. Individual EPSP/Cs were first automatically detected by MiniAnalysis Program. As bEPSP/Cs were composed of a large number of EPSP/Cs with short IEIs, we further detected individual events by using the two subjective criteria (1) their amplitude were larger than 5 S.D. of the baseline noise and (2) their 1st- and 2nd derivative were larger than 3 S.D. of the baseline noise for bEPSC and bEPSP, respectively ( Supplementary Figs S3a and S5 ). The criterion for BS was more than two consecutive spikes with <30 ms interspike interval,whereas for bEPSC it was more than three consecutive EPSCs with <20 ms IEI. We chose three events as the criterion of bEPSC because average number of EPSPs before BS/CS in current-clamp recordings was nearly three events ( Supplementary Table S1 ). Pharmacological experiments in vivo For blocking GABAergic synaptic transmission ( Supplementary Fig. S7 ), gabazine (0.4 mM in extracellular solution) was applied for 10–15 min on the brain surface before recordings. In experiments with acute harmaline ( Fig. 5a–d ) or carbenoxolone ( Supplementary Fig. S8 ) treatment, harmaline (10–30 mg kg −1 ), carbenoxolone (50 mg kg −1 ) or saline was administered intraperitoneally and recordings were performed 30 min after the injections. In experiments with chronic harmaline treatment ( Fig. 5e–h ), daily intraperitoneal injection of harmaline (30 mg kg −1 ) or saline was performed from P9 to P12, and recordings were made between P12 and P17 (ref. 31 ). In vivo two-photon Ca 2+ imaging In vivo Ca 2+ imaging was performed by using a two-photon microscope [58] (Ultima IV, Prairie Technologies) with a water-immersion objective lens (LUMPlan 40x/W/IR2, Olympus) and mode-locked Ti:sapphire laser (MaiTai, Spectra Physics). For Ca 2+ imaging experiments, pipette solution contained (in mM) 133 KMeSO 3 , 7.4 KCl, 10 HEPES, 3 Na 2 ATP, 0.3 Na 2 GTP, 0.3 MgCl 2 (pH 7.3, adjusted with KOH), 0.05 Oregon Green 488 BAPTA1 (OGB-1) and 0.05 Alexa 594. [Ca 2+ ] transients were measured using line scans at 500 Hz. The ratio of green (G: OGB-1) over red (R: Alexa 594) fluorescence was used as a measure of [Ca 2+ ]. Relative [Ca 2+ ] changes were measured as the difference between the ratio G/R (ΔG/R) before and after the onset of BS or SS simultaneously observed by current-clamp recordings. Fluorescence trace was filtered using a binominal smoothing of five points. The peak amplitude of Ca 2+ transients was defined as the difference between the baseline for 20 ms before the onset of BS or SS and the average of three points around the peak. Data were analysed using custom-written macro in IgorPro (WaveMetrics). Image stacks were obtained after recordings, and processed offline using a non-linear anisotropic diffusion filter [59] . Two-dimensional (2D) projections were performed using ImageJ ( http://rsb.info.nih.gov/ij/ ). Recordings from acute cerebellar slices Parasagittal cerebellar slices (250 μm thickness) were prepared from Sprague-Dawley rats at P4–P15 (ref. 10 ). In brief, rats were deeply anaesthetised with CO 2 and decapitated. The brain was quickly removed. Parasagittal cerebellar slices of 250 μm thickness were cut with a vibroslicer (VT1000S or 1200S; Leica) in ice-cold standard saline (see below) and kept at room temperature for at least 1 h in a submerged chamber containing standard saline that was bubbled with 95% O 2 and 5% CO 2 . A slice was then transferred to a recording chamber where it was continuously perfused with the oxygenated standard saline. Whole-cell voltage-clamp recordings were made from visually identified PC somata using an upright microscope (BX51WI, Olympus). All experiments were carried out at 32 °C. Resistance of patch pipettes were 3–6 MΩ when filled with an intracellular solution composed of (in mM): 100 CsMeSO 3 , 50 CsCl, 0.2 EGTA, 1 MgCl 2 , 2 MgATP, 0.3 Na 2 GTP, 15 HEPES, 5 QX314, pH 7.3. The pipette access resistance was compensated by 70–80%. The composition of the standard bathing solution was (in mM): 125 NaCl, 2.5 KCl, 2CaCl 2 , 1 MgSO 4 , 1.25 NaH 2 PO 4 , 26 NaHCO 3 and 20 glucose, and bubbled with 95% O 2 and 5% CO 2 . Bicuculline (10 μM) was added to block inhibitory synaptic transmission. Ionic currents were recorded with an Axopatch 1D amplifier (Molecular Devises) or EPC10 (HEKA). The signals were filtered at 3 kHz and digitized at 20 kHz using an ITC-16 interface (Instrutech). Data acquisition and offline data analysis were performed using PULSE software (HEKA). Stimuli (duration, 0.1 ms; amplitude, 0–90 V) were applied at 0.2 Hz. CFs were stimulated in the granular layer surrounding the PC soma. The number of CFs innervating the recorded PC was estimated by the number of discrete CF-EPSC steps during gradually increasing the stimulus intensity and systematically moving the stimulation pipette around the PC soma ( Supplementary Fig. S6 ) [10] . For Ca 2+ imaging experiments, pipette solution contained (in mM) 133 KMeSO 3 , 7.4 KCl, 10 HEPES, 3 Na 2 ATP, 0.3 Na 2 GTP, 0.3 MgCl 2 (pH 7.3, adjusted with KOH) and 0.05 Oregon Green 488 BAPTA1 (OGB-1). PCs were loaded for at least 10 min with the OGB-1 through patch pipettes. Fluorescence images were acquired by using a high-speed confocal laser-scanning microscope (CSU22, Yokogawa), as described [27] . Images were acquired at 30 Hz. The Ca 2+ -dependent fluorescence signals from selected regions of interest (ROI) were background-corrected and expressed as increases in fluorescence divided by the prestimulus fluorescence values (Δ F / F 0 ). The Ca 2+ signals induced by multiple-CF stimuli were obtained from primary dendritic regions. Ca 2+ imaging was conducted at 32 °C. Calculation of disparity index and disparity ratio To quantify the disparity in multiple CF-EPSCs recorded in a given PC in acute slice experiments, we calculated the disparity index (1) and disparity ratio (2) for each PC [10] . Briefly, the amplitude of individual CF-EPSC steps in a given multiply-innervated PC was measured and they were numbered in the order of their amplitudes ( A 1 , A 2 , … A i , … A N , N ≧ 2; N is the number of CFs innervating a given PC. A i is the EPSC amplitude for the CF i recorded at the same holding potential. A N represents the largest CF-EPSC). Parameters were calculated by the following equations. The disparity in bEPSCs recorded in a given PC in vivo was also quantified by calculating the disparity index and disparity ratio. First, the amplitude of individual component EPSCs in each bEPSC from a given PC were numbered in the order of their amplitudes ( A 1 , A 2 , … A i , … A N , N ≧ 3; N is the number of events in bEPSC. A N represents the largest EPSC in bEPSC). Then, the disparity index and disparity ratio were calculated for each bEPSC by the same equations used for the slice experiments. Finally, the average values of the two parameters were calculated for each PC. Statistical analysis SigmaStat (Systat Software) was used for statistical analysis. Data sets with normal distributions were tested by paired or unpaired two-tailed Student’s t -test. Non-Gaussian distributed data sets were tested by Wilcoxon signed-rank test or Mann–Whitney U –test for paired or unpaired observations, respectively. In figures, all error bars represent s.e.m. How to cite this article: Kawamura, Y. et al. Spike timing-dependent selective strengthening of single climbing fibre inputs to Purkinje cells during cerebellar development. Nat. Commun. 4:2732 doi: 10.1038/ncomms3732 (2013).